Pink marine sediments reveal rapid ice melt and Arctic meltwater discharge during Dansgaard–Oeschger warmings The climate of the last glaciation was interrupted by numerous abrupt temperature fluctuations, referred to as Greenland interstadials and stadials. During warm interstadials the meridional overturning circulation was active transferring heat to the north, whereas during cold stadials the Nordic Seas were ice-covered and the overturning circulation was disrupted. Meltwater discharge, from ice sheets surrounding the Nordic Seas, is implicated as a cause of this ocean instability, yet very little is known regarding this proposed discharge during warmings. Here we show that, during warmings, pink clay from Devonian Red Beds is transported in suspension by meltwater from the surrounding ice sheet and replaces the greenish silt that is normally deposited on the north-western slope of Svalbard during interstadials. The magnitude of the outpourings is comparable to the size of the outbursts during the deglaciation. Decreasing concentrations of ice-rafted debris during the interstadials signify that the ice sheet retreats as the meltwater production increases. During marine isotope stage 3 (MIS 3), 60–25 kyr BP, the climate of the northern hemisphere was affected by ~15 abrupt temperature fluctuations, termed Greenland interstadials and stadials. During these warmings, also known as Dansgaard–Oeschger (DO) events, temperatures over Greenland could increase more than 10 °C (ref. 1 ) just within a few years. The driving mechanisms behind the temperature shifts are still not fully understood, but injections of freshwater from the adjacent ice sheets into the North Atlantic Ocean is considered a crucial factor, as it may prevent deep-water formation and disrupt the thermohaline circulation [2] , [3] . Improved knowledge of variations in the ice sheets and in the input of freshwater to the North Atlantic Ocean in relation to the abrupt warmings is essential for a more complete understanding of the driving mechanisms [4] , [5] . Ice sheets deliver freshwater either as calving icebergs or as meltwater run-off from land. Variations in the input and distribution of icebergs are revealed by the distribution of ice-rafted debris (IRD) in marine sediments, and numerous studies have demonstrated that the production of icebergs increased during stadials and decreased during interstadials [6] , [7] . Local variations in the discharge of meltwater from land ice, however, are much more difficult to document. The best examples are from the last deglaciation, with several studies showing that rapidly deposited laminated units, widely distributed around the Nordic seas, can be dated to the Bølling interstadial and to the early Holocene. These units are thought to be the products of sediment-loaded meltwater discharge that is related to meltwater pulses Mwp-1A and Mwp-1B [8] , [9] . This study is based on a detailed investigation of core JM05-31GC, recovered from the north-western slope of Svalbard. Core JM05-31GC is one of several cores spanning a large area, with water depths ranging from 600 to 1,300 m, all of which show similar lithological changes over millennial timescales. We use changes in lithology, provenance of sediments, IRD content, planktic foraminiferal faunas, oxygen and carbon isotope values, and subsurface temperatures, calculated by transfer functions on planktic foraminifera, to estimate changes in the discharge of meltwater and in the production of icebergs in relation to DO climate shifts. The findings indicate a dynamic Svalbard ice sheet with periods of retreat (melt) and advance closely linked to the Greenland interstadials and stadials. Lithology Core JM05-31GC was retrieved from a water depth of 785 m northwest of Svalbard ( Fig. 1 ). The sediments of core JM05-31GC are varicoloured, ranging from dark green to pink and bright yellow ( Fig. 2a ). The main focus for this study is the central section between 140 and 300 cm, which consists of alternating layers of greenish-grey silt and pink (reddish-grey) clay. The pink layers are recognized in red–green spectrophotometry measurements (see Methods), which sometimes reveal faintly visible or broader peaks that can be seen with the naked eye ( Fig. 2b ). The scans also indicate that the values increase rapidly and decrease more gradually. The visible pink layers vary in thickness from 4 to 11 cm. The most prominent layers are laminated. The pink layers are similar in colour and structure to modern layers that are found in front of glaciers in fjords on north-western Svalbard and to deglacial sediments found on the inner shelf in the same area [10] , [11] , [12] ( Figs 1 and 3 ). 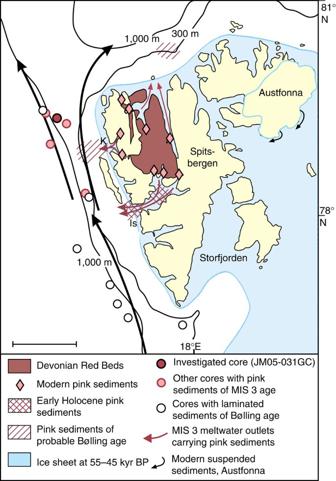Figure 1: Map of Svalbard showing distribution of Devonian Red Beds. Location of cores and distribution of meltwater deposits of Devonian provenance are indicated26. Pink diamonds and hatched areas show known distribution of pink sediments of recent, early Holocene and Bølling age on the basis of authors’ own observations and Landviket al.10, Forwicket al.11and Ó Cofaigh and Dowdeswell12. Coloured dots show locations of investigated core and other cores containing layers of pink sediments deposited during MIS 3. Open circles indicate cores containing non-pink, laminated deposits deposited during the Bølling interstadial (based on Jessenet al.22, Birgel and Hass23and Rasmussenet al.24). Brown arrows show inferred main outflow areas of pink sediment during MIS 3. Black arrows in front of Austfonna ice cap show present meltwater outflow and movement of turbid meltwater (based on Pfirman and Solheim27). The reconstructed ice margin for 55–45 ka (=early MIS 3) is based on Vorrenet al.37. IS, Isfjorden; K, Kongsfjorden. Scale bar, 100 km. Figure 1: Map of Svalbard showing distribution of Devonian Red Beds. Location of cores and distribution of meltwater deposits of Devonian provenance are indicated [26] . Pink diamonds and hatched areas show known distribution of pink sediments of recent, early Holocene and Bølling age on the basis of authors’ own observations and Landvik et al. [10] , Forwick et al. [11] and Ó Cofaigh and Dowdeswell [12] . Coloured dots show locations of investigated core and other cores containing layers of pink sediments deposited during MIS 3. Open circles indicate cores containing non-pink, laminated deposits deposited during the Bølling interstadial (based on Jessen et al. [22] , Birgel and Hass [23] and Rasmussen et al. [24] ). Brown arrows show inferred main outflow areas of pink sediment during MIS 3. Black arrows in front of Austfonna ice cap show present meltwater outflow and movement of turbid meltwater (based on Pfirman and Solheim [27] ). The reconstructed ice margin for 55–45 ka (=early MIS 3) is based on Vorren et al. [37] . IS, Isfjorden; K, Kongsfjorden. Scale bar, 100 km. 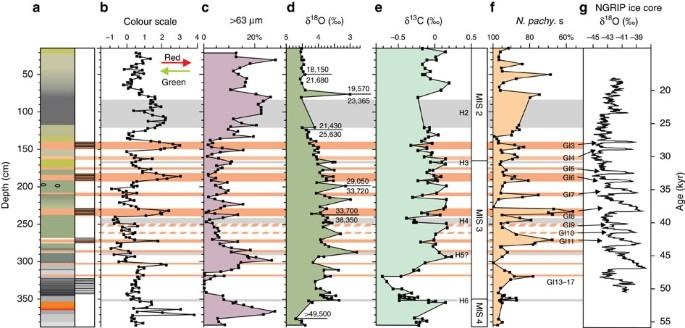Figure 2: Comparison of JM05-31GC sediment logs and climate with the NGRIP ice core. The records comprise the time period 20,000–55,000 years BP. (a) Lithological log showing colour variations of sediments and distribution of laminated layers. (b) Spectrophotometer data showing red–green spectrum. (c) Weight percentage of grains >63 μm. (d) Planktic δ18O values measured onN. pachydermas. Dated samples are indicated.14C ages are shown above marker lines, calibrated ages are shown below marker lines. (e) Planktic δ13C values measured onN. pachydermas. Heinrich event (H) numbers are indicated. (f) Relative abundance of planktic foraminiferaN. pachydermas (>100 μm). Greenland interstadial (GI) numbers are indicated. (g) δ18O record measured on NGRIP ice core on the GICC05 timescale before 2,000 years (data from Svenssonet al.20). Pink horizontal bars mark pink sediment layers. Pink dashed bars mark layers only indicated in the red–green colour scale. Grey horizontal bars mark Heinrich events. Marine isotope stages (MIS) are indicated. Full size image Figure 2: Comparison of JM05-31GC sediment logs and climate with the NGRIP ice core. The records comprise the time period 20,000–55,000 years BP. ( a ) Lithological log showing colour variations of sediments and distribution of laminated layers. ( b ) Spectrophotometer data showing red–green spectrum. ( c ) Weight percentage of grains >63 μm. ( d ) Planktic δ 18 O values measured on N. pachyderma s. Dated samples are indicated. 14 C ages are shown above marker lines, calibrated ages are shown below marker lines. ( e ) Planktic δ 13 C values measured on N. pachyderma s. Heinrich event (H) numbers are indicated. ( f ) Relative abundance of planktic foraminifera N. pachyderma s (>100 μm). Greenland interstadial (GI) numbers are indicated. ( g ) δ 18 O record measured on NGRIP ice core on the GICC05 timescale before 2,000 years (data from Svensson et al. [20] ). Pink horizontal bars mark pink sediment layers. Pink dashed bars mark layers only indicated in the red–green colour scale. Grey horizontal bars mark Heinrich events. Marine isotope stages (MIS) are indicated. 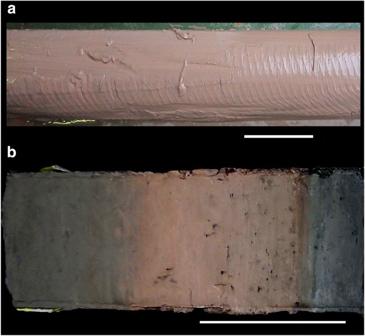Figure 3: Pink sediments from the western margin of Svalbard. (a) Holocene pink sediments from the inner part of Kongsfjorden (in front of Kongsvegen Glacier). (b) Pink sediment layer referred to Bølling interstadial from Kongsfjorden Trough on the shelf outside of Kongsfjorden. Scale bar, 10 cm. Full size image Figure 3: Pink sediments from the western margin of Svalbard. ( a ) Holocene pink sediments from the inner part of Kongsfjorden (in front of Kongsvegen Glacier). ( b ) Pink sediment layer referred to Bølling interstadial from Kongsfjorden Trough on the shelf outside of Kongsfjorden. Scale bar, 10 cm. Full size image Age and stratigraphy The AMS 14 C dates in combination with the δ 18 O record demonstrate that core JM05-31GC comprises marine isotope stages MIS 4–MIS 2 ( Fig. 2 and Table 1 ). Three AMS 14 C dates and overall high isotope values indicate that the greenish-grey sediments in the upper part of the core, above 140 cm, can be referred to MIS 2 ( Fig. 2d and Table 1 ). The alternating red–green-coloured deposits between 125 and 320 cm are referred to MIS 3 on the basis of two AMS 14 C dates and the highly variable δ 18 O values. Fluctuating isotope values are characteristic of MIS 3 in the North Atlantic and Nordic Seas areas [6] , [13] , [14] . The lower part of the core, below c. 320 cm, has only a few δ 18 O measurements, and the AMS 14 C date is infinite ( Fig. 2d and Table 1 ). This part probably correlates with MIS 4 (354–376 cm) and the MIS 4–MIS 3 transition (354–320 cm). The sediments here are a homogeneous bluish grey layer, except for a sandy yellowish layer and a laminated deposit between c. 320 and 345 cm ( Fig. 2a ). Similar laminated deposits have been described from several cores from the Svalbard margin and are typical of the MIS 4–MIS 3 transition [13] , [14] , [15] . Core JM05-031GC thus covers the time interval c. 70–18 kyr BP. Table 1 AMS 14 C dates and calibrated ages of JM05-031GC. Full size table Identification of DO events and correlation of pink layers Core JM05-31GC is faunistically and isotopically very similar to previously published cores LINK16 and ENAM93-21 from the SE Norwegian Sea [16] , [17] . LINK16 and ENAM93-21 have been correlated to the Greenland NGRIP ice core timescale in great detail, and in both cores all Greenland interstadials and stadials from MIS 2 to MIS 4 have been identified. Stadials and Heinrich events are characterized by low planktic δ 18 O and δ 13 C values, high percentages of the planktic foraminiferal species Neogloboquadrina pachyderma sinistral (s) and high concentrations of IRD (grains >63 μm) ( Fig. 2 ). Heinrich event H6 is particularly prominent because of unusually low δ 18 O and δ 13 C values [6] , [18] , [19] ( Fig. 2 ). Interstadials are characterized by generally high δ 18 O and δ 13 C values and lower percentages of N. pachyderma s and IRD. The great similarity between JM05-031GC, LINK16 and ENAM93-21 and the close correlation to the NGRIP ice core allow us to identify Heinrich events H6–H2 ( Fig. 2 ). Within the section of highest resolution, from 125 to 280 cm, we have identified Greenland interstadials 11–3 ( Fig. 2 ). The correlation shows that the pink layers in JM05-031GC correspond to the interstadials, whereas the greenish-grey layers correspond to the stadials. Interstadials 10 and 9 are only discernible in the red–green colour record and were not detected during the initial visual description of the core. Construction of an age model We have constructed an age model for the interval 125–280 cm on the basis of the calibrated AMS 14 C dates, and the assumption that sedimentation rates between dated points were linear ( Figs 4 and 5 ). 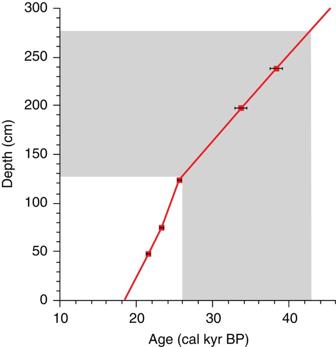Figure 4: Age–depth model for JM05-31GC based on calibrated14C ages. 1σ error bars are marked for each dating point. Grey area indicates the core section investigated in this study. Figure 4: Age–depth model for JM05-31GC based on calibrated 14 C ages. 1σ error bars are marked for each dating point. Grey area indicates the core section investigated in this study. 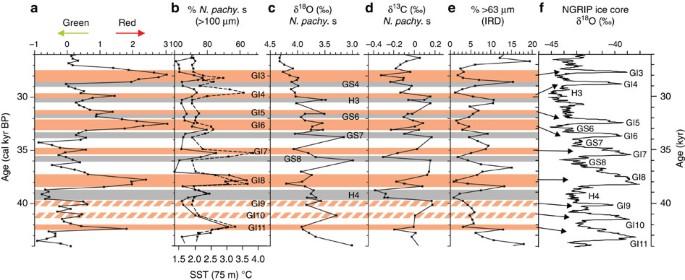Figure 5: Greenland interstadial events 11–3 in core JM05-31GC versus the NGRIP ice core. (a) Spectrophotometer data showing red–green spectrum. (b) Relative abundance of planktic foraminiferaN. pachydermas >100 μm (solid line) and subsurface temperatures (SST) (75 m) estimated by transfer functions from census counts of planktic foraminifera species >150 μm (dashed line). Greenland interstadial (GI) numbers are indicated. (c) Planktic δ18O values measured onN. pachydermas. Heinrich event (H) and stadial (GS) numbers are indicated. (d) Planktic δ13C values measured onN. pachydermas. (e) Weight percentage of grains >63 μm. (f) δ18O values measured on NGRIP ice core on the GICC05 timescale before 2,000 years (data from Svenssonet al.20). Greenland interstadial (GI), stadial (GS) and Heinrich event (H) numbers are indicated. Pink horizontal bars mark pink layers. Dashed horizontal bars mark layers only indicated by the red–green colour scale. Grey horizontal bars mark Heinrich events and Greenland stadials. Full size image Figure 5: Greenland interstadial events 11–3 in core JM05-31GC versus the NGRIP ice core. ( a ) Spectrophotometer data showing red–green spectrum. ( b ) Relative abundance of planktic foraminifera N. pachyderma s >100 μm (solid line) and subsurface temperatures (SST) (75 m) estimated by transfer functions from census counts of planktic foraminifera species >150 μm (dashed line). Greenland interstadial (GI) numbers are indicated. ( c ) Planktic δ 18 O values measured on N. pachyderma s. Heinrich event (H) and stadial (GS) numbers are indicated. ( d ) Planktic δ 13 C values measured on N. pachyderma s. ( e ) Weight percentage of grains >63 μm. ( f ) δ 18 O values measured on NGRIP ice core on the GICC05 timescale before 2,000 years (data from Svensson et al. [20] ). Greenland interstadial (GI), stadial (GS) and Heinrich event (H) numbers are indicated. Pink horizontal bars mark pink layers. Dashed horizontal bars mark layers only indicated by the red–green colour scale. Grey horizontal bars mark Heinrich events and Greenland stadials. Full size image The calculated ages for the identified interstadials and stadials in core JM05-31GC differ slightly from the ice core ages for the same events [20] , in particular in the upper part of the investigated interval ( Fig. 5e,f ). These discrepancies may be due to the use of benthic material in some of the AMS 14 C datings ( Table 1 ). It has been shown that benthic material may enhance or diminish the reservoir age as compared with planktic dates [21] . However, it is more likely that the differences are primarily caused by frequent changes in sedimentation rate. Several studies have shown that the sedimentation rate on the Svalbard margin was low during Heinrich event H1 and very high during the following Bølling interstadial [13] , [22] , [23] , [24] , [25] . It seems probable that similar differences occurred between the stadials and interstadials studied here. This indicates that the pink interstadial layers represent shorter time periods and the stadials longer time periods than indicated in Fig. 5 . The average time span for the deposition of the pink layers, calculated on the basis of the age model, is close to 600 years, ranging from 380 to 1,150 years, but because of the possible elevated sedimentation rates the actual durations were probably less. Overall, the differences between the ages recorded in JM05-31GC and the ice core ages seem relatively small (<1,000 years) ( Fig. 5e,f ), and close to the error of the calibrated ages and the error of the NGRIP timescale [20] . In both the marine core and the NGRIP ice core, the dating error is 700–900 years for the time interval between 35,000 and 44,000 ice core years BP. Today, pink sediments are deposited in the inner fjords of north-western Spitsbergen, the largest island in the Svalbard archipelago [10] , [11] . The highest concentrations are found close to the glaciers that drain from the interior of the island, for example, in Isfjorden in front of the Tunabreen glacier [11] and in Kongfjorden in front of the Kongsvegen and Kronebreen glaciers [12] ( Fig. 1 ). The provenance of the pink sediments is the Devonian Red Beds, which constitute the largest exposed geologic formation on north-western Spitsbergen [26] ( Fig. 1 ). The sediments are generally carried by meltwater into the fjords via submarine glacial conduits [12] . The meltwater rises to the surface, and the red-coloured fraction spreads over the inner parts of the fjords in sediment-laden meltwater suspension plumes [11] , [12] . Nearly all the suspended material is deposited within a few kilometres of the outlet [27] . Several observations have shown that sediments settling from meltwater plumes (plumites) are often laminated and deposited at high sedimentation rates [12] , [22] , [28] , [29] . The great lithological similarity between the modern pink fjord sediments and the pink layers in core JM05-031GC indicates that they have the same provenance and were deposited under similar circumstances. The pink sediments are thus thought to have originated from the Devonian Red Beds on Spitsbergen, and thus transported to the slope by glacial meltwater plumes. The pink layers clearly signify increased melting of the Svalbard ice sheet, which is in good agreement with their stratigraphic position. The pink layers correlate, as noted above, with interstadials, which, in the Nordic seas, are characterized by high subsurface temperatures, low relative abundance of the polar planktic foraminiferal species N. pachyderma s, low concentrations of IRD and high δ 18 O and δ 13 C values ( Fig. 5 ). Within the best preserved interval, comprising Greenland interstadials 11–3, all warming events are represented by a pink layer ( Fig. 5a,b ). It is thought that, during this interval, the warmer atmosphere during the interstadials increased the melting rate of the ice sheets. The relatively low content of IRD in the pink layers in comparison to the greenish-grey mud in-between indicates that the production of icebergs decreased, and the ice margin retreated as the production of meltwater increased. The large meltwater production during interstadials seems contradictory to the higher δ 18 O values seen in most pink layers ( Fig. 5c ). However, it appears that N. pachyderma s generally only picks up meltwater signals and records low δ 18 O values when the meltwater is from icebergs [30] . Icebergs can generate a >150 m thick surface layer of polar meltwater similar to the stratified upper layers found in the modern Arctic Ocean, where N. pachyderma s displays low δ 18 O values [31] . Even the well-documented huge meltwater discharge that occurred during the Bølling interstadial is not reflected in the δ 18 O values of the Nordic Seas, and the meltwater layer must have been much thinner, [18] , [22] , [23] as N. pachyderma s normally lives at water depths between 100 and 200 m (ref. 32 ). The δ 13 C record of JM05-031GC resembles a record from the NE Atlantic Ocean [33] . The high values during interstadials are interpreted to indicate improved ventilation in comparison to the stadials and Heinrich events, where low values indicate surface stratification [33] . The widespread distribution of the pink interstadial deposits indicates that the glacial conditions during MIS 3 were very different from the present situation, where pink deposits are confined to the inner fjords. The size of the ice sheet during MIS 3 is uncertain, but it was undoubtedly larger than that today, with the ice margin being closer to the coastline with an open marine ice front (see below) ( Fig. 1 ). The best modern analogue from Svalbard to the situation during MIS 3 is probably Austfonna Ice Cap on Nordaustlandet, which also has an open marine ice front ( Fig. 1 ). The sediment-laden meltwater from Austfonna is carried away from the outflow conduits by costal currents and can be followed at the surface in a 10 km wide zone along the coast for up to 60 km (ref. 27 ). Still, the discharge from Austfonna seems much too small when compared with the situation during MIS 3, when the distance from the core site to the major outflows at Kongsfjorden and Isfjorden is estimated to have been c. 100 and 200 km, respectively, and the shortest distance to the ice margin was c. 90 km ( Fig. 1 ). The outflows during MIS 3 can probably best be compared with the outflow during the Bølling interstadial at the beginning of the deglaciation c. 14.5 kyr BP, when a 10 cm to more than 2 m thick laminated bed was deposited along the western margin of Svalbard over a time span of less than 400 years [23] , [24] , [28] , [33] , which is comparable to the estimated duration of the melting events during MIS 3 (see above). The bed is found at distances from the ice margin that are comparable to the distance from our core site to the ice margin during MIS 3. The laminated layer from Bølling is apparently only pink in records from shelf areas [10] ( Fig. 1 ). In the slope records and south of Isfjorden, the layer is bluish grey, indicating a more southern sediment provenance. The laminated layer is synchronous with rapidly deposited sediments from the eastern margin of Svalbard [34] , the western margin of Norway and the Faroe Islands [15] . This meltwater discharge coincides with meltwater pulse Mwp-1A [8] , which has been dated to 14.6–14.3 kyr BP [8] , [9] , [35] . The early Holocene meltwater pulse Mwp-1B is also associated with laminated layers, although these layers seem to cover a smaller area compared with the layer linked to Mwp-1A, indicating that this melting event was smaller [8] , [11] ( Fig. 1 ). It should finally be noted that the thickest and the most prominent laminated bed in JM05-031GC occurs from 329 to 345 cm, immediately above Heinrich event H6 ( Fig. 2a ) and follows the same sequence of events as the Bølling interstadial and Heinrich event H1 (ref. 13 ). Off Svalbard, pink layers from MIS 3 are absent in the cores from south of Isfjorden [22] due to the lack of Devonian Red Beds on this part of Spitsbergen ( Fig. 1 ). The interstadial sediments here consist of greenish-grey deposits similar to the stadial deposits, leaving no visible sign of variations in the input of meltwater. Nevertheless, we must assume that the ice sheet reacted in the same way all along the western margin of the Svalbard–Barents Sea margin. In fact, the wide distribution and similarity of the laminated sediments deposited during the Bølling interstadial suggests that the Scandinavian ice sheet reacted almost synchronously with the Svalbard–Barents Sea ice sheet [28] , [36] . The glacial record of Svalbard during MIS 3 is very fragmentary, but it appears that the major ice sheet movements followed the pattern of the better-documented Scandinavian ice sheet [37] . During MIS 4, c. 70–60 kyr BP, the Barents–Kara Sea (including Svalbard) and Scandinavia were covered by a huge confluent ice sheet [37] , [38] , [39] , [40] , [41] . The glaciation was followed by a rapid deglaciation, and from c. 55 to 25 kyr BP, the ice sheets on Svalbard and Scandinavia were apparently separated by an ice-free Barents Sea [37] , [40] , [41] . During the warmest period of MIS 3, 40–35 kyr BP, the Scandinavian ice sheet was most likely limited to the central part of Norway and Sweden [39] , [41] . From c. 32 kyr BP the ice sheets expanded, and from c. 25 kyr BP Svalbard and Scandinavia were once again covered by a continuous ice sheet [37] , [39] . The poor record from Svalbard does not allow any detailed reconstructions of the ice sheet during MIS 3 (ref. 42 ). From c. 55–45 kyr BP, the western ice margin seems to have been close to the present coastline [37] . During the mildest part of MIS 3 the ice sheet retreated inland, and during warm spikes the islands may periodically have been ice free [37] . New data from Norway [43] , [44] , [45] , Sweden and Finland [46] , [47] indicate that the Scandinavian ice sheet during MIS 3 was more dynamic than previously recognized. The evidence is lacking in temporal resolution, but two rapid advances beyond the coastline of Norway seem well-documented [39] , [40] , [43] . The first advance is correlated with Greenland interstadial 10 and dated to ~41 kyr BP on the GICC05 timescale. The second advance is correlated with Greenland stadial 7 and dated to c. 34.5 kyr BP. The intervening period includes the Ålesund interstadial, which has been correlated with the period corresponding to Greenland interstadials GI8–GI7 (38.2–34.5 kyr BP on the GICC05 timescale) [39] , [45] . The evidence presented in the present paper reveals a dynamic Svalbard ice sheet with a repeated shift, on a millennium timescale, between warm interstadials characterized by melting, retreating ice and a strong outpouring of meltwater, and cold stadials characterized by a growing ice sheet, increased production of icebergs and IRD. Considering the evidence from Norway, it seems probable that during each interstadial, the ice margin retreated inland well behind the coastline. The minimum extent of the ice sheet is uncertain, but it was probably always larger than at present. During interstadial–stadial transitional periods, the ice sheet probably advanced beyond the coastline onto the shelf, comparable with the development during cold events in Norway. From 32 to 30 kyr BP, the Eurasian ice sheets started to expand again [37] , [39] . The surprising thickness of the pink layer correlated with Greenland interstadial GI3 ( Fig. 5a ) might indicate that the ice front at c. 28 kyr BP was closer to the core site and thus to the shelf edge than that observed during the earlier advances. Broecker et al. [2] hypothesized, in their salt–oscillator model for the DO temperature shifts, that under warm interstadial conditions the land-based ice would discharge meltwater into the North Atlantic. This would result in cooling and freshening of the surface water and a weaker deep-water formation. The ice sheets and the sea ice would then start to grow again eventually, slowing the meridional overturning circulation. The record of core JM05-31GC provides crucial evidence for efforts to understand this instability, as it confirms some of the fundamental assumptions in the salt–oscillator model. Most importantly, the record corroborates that during the warm interstadials, large amounts of meltwater were released from the ice sheets along the north-eastern margin of the Nordic seas ( Fig. 6a ). The record also indicates that the ice margin retreated as the meltwater production increased. In agreement with the model, we observe decreasing temperatures and rapidly increasing ice rafting in the layers immediately above the meltwater deposits ( Fig. 6b ). Finally, as the cold stadial conditions progressed, the concentration of IRD decreased, indicating reduced ice rafting and the establishment of a permanent sea ice cover [25] ( Fig. 6c ). 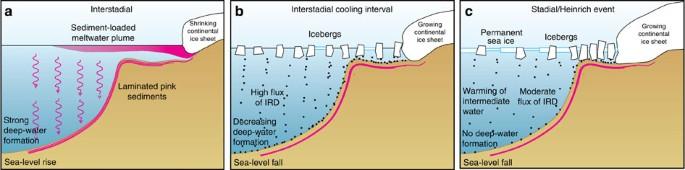Figure 6: Schematic reconstruction of land and sea ice conditions at core site JM05-031GC. (a) Peak interstadial warm phase with discharge of turbid, reddish meltwater from land-based ice sheets and fallout of pink sediments (pink wavy arrows). (b) Cooling phase of the interstadial intervals showing growing ice sheet, increased iceberg calving and high production of ice-rafted debris (IRD). (c) Cold stadial/Heinrich event with some ice rafting and near-permanent sea ice cover, and concurrent warming at intermediate depth18. Figure 6: Schematic reconstruction of land and sea ice conditions at core site JM05-031GC. ( a ) Peak interstadial warm phase with discharge of turbid, reddish meltwater from land-based ice sheets and fallout of pink sediments (pink wavy arrows). ( b ) Cooling phase of the interstadial intervals showing growing ice sheet, increased iceberg calving and high production of ice-rafted debris (IRD). ( c ) Cold stadial/Heinrich event with some ice rafting and near-permanent sea ice cover, and concurrent warming at intermediate depth [18] . Full size image Our results also have implications for the understanding of the rapid sea-level changes that occurred on millennial timescales during MIS 3. The magnitude of these changes is generally estimated to range from 20 to 30 m (ref. 48 ). However, there is considerable uncertainty as to their timing and source. Some studies indicate that the main sea-level rises occurred during the stadials and the source was Antarctica [48] ; others indicate equal contributions from both hemispheres [49] or mainly from a northern source [50] , [51] . In this study, we have established the precise chronology for eight major meltwater discharges during MIS 3, involving the Svalbard–Barents Sea ice sheet and probably also the Scandinavian ice sheet. The present study provides clear evidence of a significant northern component to the millennial timescale sea-level changes. Our observations also support emerging evidence of a much more dynamic Eurasian ice sheet than previously recognized, with retreat and advance closely linked to the Greenland interstadials and stadials [39] , [40] . Core logging The core was collected in 2005 from a water depth of 785 m on the north-western slope of Svalbard. The 376 cm long core was split into two halves, and one half of the core was X-rayed. The core was visually described, and sediment colour was determined using the Munsell Soil Colour Chart. Thereafter, the colour of the sediment was measured every 2 cm using a Colortron Spectrophotometer [52] , following the laboratory designations of the Commission Internationale de l’Eclairage (CIE). The X-ray photos revealed that the thicker and the most prominent pink layers were laminated. Faunal analysis The core was sampled in 0.7 cm thick slices taken at 1, 2 or 3 cm intervals except for the upper part, where it was sampled every 5 cm. The samples were weighed and dried at 50 °C and weighed again. The samples were sieved over mesh sizes 63 and 100 μm, and the residues were dried and weighed. The residues >100 μm were spread evenly over a picking tray, and ~300 planktic foraminiferal specimens were counted and identified up to species level. In certain intervals, the number of planktic foraminifera was too low for quantification. The samples were subsequently dry sieved over mesh size 150 μm, and the planktic foraminifera were re-counted for calculations of absolute temperatures (see below). Temperature calculations Summer sea-surface water temperatures (°C) were estimated by transfer functions using the C2 program [53] . The calculations were based on the 150 μm size fraction of planktic foraminifera. We applied the WAPLS (weighed average partial least-squares) method using three components, following the recommendations of Birks [54] . The MARGO database [55] , [56] , [57] together with temperatures from the World Ocean Atlas (2009) [58] were used for the calculations. The summer temperatures were calculated for 75 m water depth. This water depth represents the average water depth at which the planktic foraminiferal species live [32] . Isotope analyses and dating Stable isotope measurements were performed on the planktic foraminiferal species N. pachyderma s at Woods Hole Oceanographic Institution [59] . Pristine specimens of similar size (around 200 μm), square shape and with four chambers were picked. Several intervals could not be measured because of too low availability of pristine shells. AMS 14 C dates were performed at the AMS Dating Centre at the University of Aarhus, Denmark, on specimens of N. pachyderma s, bivalves and benthic foraminiferal assemblages ( Table 1 ). The conventional AMS dates were calibrated to calendar ages using the Calib 6.01 program and the Marine09 calibration data, which operates with a standard reservoir correction of −405 years for sediments older than 12.5 cal kyr BP [60] , [61] . The mid-point value from the calibrated age range ±1 σ was used (95% confidence level) ( Table 1 ). How to cite this article: Rasmussen, T. L. and Thomsen, E. Pink marine sediments reveal rapid ice melt and Arctic meltwater discharge during Dansgaard–Oeschger warmings. Nat. Commun. 4:2849 doi: 10.1038/ncomms3849 (2013).